Early dynamic fate changes in haemogenic endothelium characterized at the single-cell level Haematopoietic stem cells (HSCs) are the founding cells of the adult haematopoietic system, born during ontogeny from a specialized subset of endothelium, the haemogenic endothelium (HE) via an endothelial-to-haematopoietic transition (EHT). Although recently imaged in real time, the underlying mechanism of EHT is still poorly understood. We have generated a Runx1 +23 enhancer-reporter transgenic mouse (23GFP) for the prospective isolation of HE throughout embryonic development. Here we perform functional analysis of over 1,800 and transcriptional analysis of 268 single 23GFP + HE cells to explore the onset of EHT at the single-cell level. We show that initiation of the haematopoietic programme occurs in cells still embedded in the endothelial layer, and is accompanied by a previously unrecognized early loss of endothelial potential before HSCs emerge. Our data therefore provide important insights on the timeline of early haematopoietic commitment. Definitive haematopoietic progenitors and long-term haematopoietic stem cells (HSCs) are thought to originate during ontogeny from a specialized subset of endothelium, so-called haemogenic endothelium (HE) [1] , [2] , [3] , [4] . Arguably the strongest support for the endothelial origin of haematopoietic cells comes from recent time-lapse imaging studies that directly visualized the transition of endothelium into blood, both in vitro [5] and in / ex vivo [6] , [7] , [8] , [9] . What has remained unclear, however, is at what stage during this endothelial-to-haematopoietic transition (EHT) cells actually change their fate and initiate the process of commitment to the haematopoietic lineage, and how this fate change is regulated at the molecular level. Addressing these and other questions will be critical to obtain a better understanding of the cellular hierarchies and the signalling and transcription factor gene regulatory networks that underlie the specification of definitive hematopoietic stem and progenitor cells. This in turn will inform the rational development of future regenerative therapies involving the efficient generation of definitive HSCs from embryonic stem cells, induced pluripotent cells or via direct reprogramming, which at present has not been possible [10] , [11] , [12] , [13] , [14] , [15] , [16] . A major hurdle in dissecting the process of EHT has been the lack of positive fluorescent markers specific for haemogenic, but not non-haemogenic, endothelium. To obtain such a marker, we have initiated studies into the regulation of the transcription factor Runx1 , which is expressed during, and critically required for EHT [7] , [8] , [9] , [11] , [17] , [18] , [19] , [20] . We recently identified the Runx1 +23 haematopoietic enhancer and generated transgenic mouse lines carrying a LacZ or Gfp reporter gene transcribed from the hsp68 minimal promoter under the spatiotemporal control of the Runx1 +23 enhancer [21] , [22] . In these lines, reporter gene expression recapitulates endogenous Runx1 expression in haematopoietic sites only, where +23-mediated reporter gene expression is comparable with expression from a Runx1-LacZ knock-in allele [22] . Indeed, functional assays showed that +23 enhancer-reporter expression marked most, if not all, of the emerging haematopoietic stem and progenitor cells, similar to endogenous Runx1 [21] , [22] . Importantly, we never observed reproducible +23-mediated reporter gene expression in the non-haematopoietic embryonic sites of endogenous Runx1 expression, indicating the haematopoietic specificity of the +23 enhancer [22] . In the present study, we establish that +23 enhancer-mediated GFP expression (referred to as 23GFP throughout) prospectively labels all haematopoietic-fated endothelial cells. Comprehensive functional analysis of 1,800 single 23GFP + haemogenic endothelial cells and transcriptional analysis of 268 single 23GFP + haemogenic endothelial cells reveals that HE is itself highly transitory, initiating dynamic changes towards a haematopoietic fate earlier than previously recognized, two days before HSCs emerge, while cells are still part of the endothelial wall. Furthermore, initiation of the haematopoietic differentiation programme is accompanied by a previously unrecognized early loss of endothelial potential. The 23GFP transgene marks a subset of embryonic endothelium To obtain a positive fluorescent marker for haemogenic endothelium, we generated a transgenic reporter mouse line in which the +23 enhancer of the haematopoietic master regulator Runx1 mediates the expression of GFP specifically to the haemogenic/haematopoietic sites of the developing embryo, in a spatiotemporal pattern similar to the haematopoietic expression of a Runx1-LacZ knock-in allele [21] , [22] ; ( Supplementary Fig. S1a–d ). In these 23GFP transgenic embryos, GFP was shown to mark functionally defined haematopoietic stem and progenitor cells [21] . Non-haematopoietic sites of Runx1 expression are not marked by the +23 enhancer [22] , indicative of its haematopoietic specificity. Here, we further characterized the expression of the reporter-enhancer transgene in haemogenic sites by immunostaining for VE-Cadherin (VE-Cadh) expression. In addition to its reported expression in haematopoietic cells [21] , [22] , 23GFP expression was detected in a subset of VE-Cadh + endothelial cells (ECs) of the (paired) dorsal aorta(e) in the para-aortic splanchnopleura (PAS)/aorta-gonad-mesonephros (AGM) region, the vitelline and umbilical (VU) arteries, and the yolk sac vasculature ( Fig. 1a ; Supplementary Fig. S1e,f ). 23GFP expression was also observed in placental vessels ( Supplementary Fig. S1g ) [22] . In this study, we mainly focused on the haemogenic sites known to autonomously generate HSCs: the PAS/AGM and VU arteries [23] , [24] , [25] that contain a definitive type HE [26] , [27] . In the PAS, 23GFP expression was already prevalent in the endothelium of the paired dorsal aortae at embryonic day (E) 8–8.5, when Runx1-LacZ expression commences [22] , and before endogenous Runx1 protein expression could be detected by immunofluorescence (starting laterally in the dorsal aorta from ~23 somite pairs (sp)/E9.25; Fig. 1b ). The absence of other Runx1 regulatory elements and/or the lack of Runx1- specific posttranscriptional regulation could underlie the differences in onset of expression of the 23GFP reporter and endogenous Runx1. To examine whether the early onset of 23GFP in ECs reflects a biologically distinct subset, we performed genome-wide expression profiling of E8.5 23GFP + and 23GFP − ECs, along with the first emerging CD41 + haematopoietic progenitor cells (HPCs; Fig. 1c ). 23GFP + and 23GFP − ECs were stringently gated as VE-Cadh + Ter119 − CD45 − CD41 − , and CD41 + HPC as 23GFP + VE-Cadh + Ter119 − CD45 − CD41 + cells ( Supplementary Fig. S1h ). Hierarchical clustering of the expression data revealed that E8.5 23GFP + ECs have a distinct transcriptional signature closer to the first emerging CD41 + HPCs than to the 23GFP − endothelium ( Fig. 1d ). Five hundred and sixteen annotated genes were differentially expressed between the 23GFP + and 23GFP − ECs, including 45 transcription factors and 11 endothelial junction genes ( Supplementary Data 1 ). The top differentially affected gene ontology processes overrepresented in 23GFP + ECs (green bars, Fig.1e ) included genes associated with angiogenesis and cell migration, indicative of an active endothelial nature, and interestingly also genes expressed in response to estradiol, which was recently implicated in the formation of the hematopoietic system [28] . In conclusion, 23GFP expression is detected in a specific subset of the endothelium that precedes and later overlaps with endogenous Runx1 protein expression, suggesting that the 23GFP transgene prospectively identifies the HE. 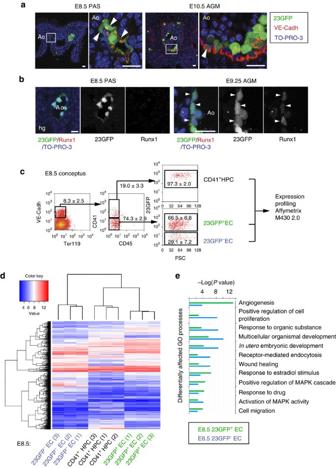Figure 1:TheRunx1+23 haematopoietic-specific enhancer marks a distinct subset of endothelium in mouse haemogenic sites. (a) VE-Cadh immunostaining (red) and 23GFP transgene expression (green) in 10 μm cryosections through the posterior region of E8.5 (7–10 sp) and E10.5 (31–34 sp) 23GFP transgenic embryos. Nuclear stain (TO-PRO-3) in blue. Higher magnification images of the boxed areas show co-expression of VE-Cadh and 23GFP. Arrowhead: example of 23GFP expression in VE-Cadh+endothelial cells. Scale bar, 20 μm. (b) Merged and single channel images of Runx1 immunohistochemistry on 23GFP expressing sections of E8.5 (10 sp) and E9.25 (23 sp). Arrowhead: 23GFP and Runx1 co-expression, asterisk: Runx1 but no 23GFP expression. Ao, dorsal aorta; Hg, hind gut; Vit, vitelline artery; scale bar, 20 μm. (c) Flow cytometric analysis further corroborates 23GFP expression in E8.5 (4–12 sp) VE-Cadh+Ter119−CD45−CD41−endothelial cells. Representative dot plots and mean percentages±s.d. are from three independent analyses of pooled tissues. Sort gates are indicated. (d) Hierarchical clustering and heatmap of whole-genome gene expression data (Affymetrix) from 23GFP+and 23GFP−VE-Cadh+Ter119−CD45−CD41−EC and 23GFP+VE-Cadh+Ter119−CD45−CD41+HPC. Numbers in parentheses indicate the biological sample. There are 516 unique annotated probe IDs differentially expressed between 23GFP+and 23GFP−ECs (seeSupplementary Data 1for the full list). The top differentially affected GO processes overrepresented in this list are shown in (e). Figure 1: The Runx1 +23 haematopoietic-specific enhancer marks a distinct subset of endothelium in mouse haemogenic sites. ( a ) VE-Cadh immunostaining (red) and 23GFP transgene expression (green) in 10 μm cryosections through the posterior region of E8.5 (7–10 sp) and E10.5 (31–34 sp) 23GFP transgenic embryos. Nuclear stain (TO-PRO-3) in blue. Higher magnification images of the boxed areas show co-expression of VE-Cadh and 23GFP. Arrowhead: example of 23GFP expression in VE-Cadh + endothelial cells. Scale bar, 20 μm. ( b ) Merged and single channel images of Runx1 immunohistochemistry on 23GFP expressing sections of E8.5 (10 sp) and E9.25 (23 sp). Arrowhead: 23GFP and Runx1 co-expression, asterisk: Runx1 but no 23GFP expression. Ao, dorsal aorta; Hg, hind gut; Vit, vitelline artery; scale bar, 20 μm. ( c ) Flow cytometric analysis further corroborates 23GFP expression in E8.5 (4–12 sp) VE-Cadh + Ter119 − CD45 − CD41 − endothelial cells. Representative dot plots and mean percentages±s.d. are from three independent analyses of pooled tissues. Sort gates are indicated. ( d ) Hierarchical clustering and heatmap of whole-genome gene expression data (Affymetrix) from 23GFP + and 23GFP − VE-Cadh + Ter119 − CD45 − CD41 − EC and 23GFP + VE-Cadh + Ter119 − CD45 − CD41 + HPC. Numbers in parentheses indicate the biological sample. There are 516 unique annotated probe IDs differentially expressed between 23GFP + and 23GFP − ECs (see Supplementary Data 1 for the full list). The top differentially affected GO processes overrepresented in this list are shown in ( e ). Full size image 23GFP + endothelial cells are haemogenic HE has been defined as cells with an endothelial morphology and phenotype ( cf . Fig. 1a,c ) that form endothelial tubules in culture and are competent to generate haematopoietic progeny [29] , [30] . To examine the haemogenic potential of the 23GFP + endothelium, 23GFP + and 23GFP − VE-Cadh + Ter119 − CD45 − CD41 − endothelial cells (EC) were isolated from the E8.5 conceptus as before and from the E10.5 AGM+VU ( Supplementary Fig. S2b,c ) and cultured in bulk on OP9 stroma [31] in conditions supporting the generation of haematopoietic progeny. Consistently, only the 23GFP + endothelium, and never the 23GFP − endothelium, gave rise to haematopoietic progeny, generating both myeloid and lymphoid cells, ( Fig. 2a–d ; Supplementary Fig. S2d ). Haemogenic potential of the 23GFP + endothelium was more robust at E10.5 than at E8.5 ( Fig. 2b ), an observation further supported by limiting dilution experiments of 23GFP + endothelium at E9.5 and E10.5 ( Supplementary Fig. S2e ). Similar results were obtained from 23GFP + and 23GFP − yolk sac endothelium ( Supplementary Fig. S2f ). Importantly, no significant haematopoietic clonogenic potential, indicative of the presence of HPCs rather than HE, was detected in the 23GFP + endothelial population ( Supplementary Fig. S2g ). In summary, these results show that throughout development, haemogenic potential segregates with the 23GFP + endothelium, allowing for the prospective isolation of cells fated to undergo EHT. 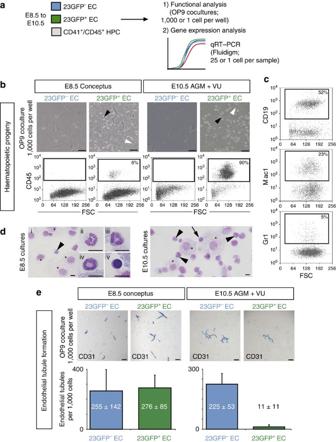Figure 2:Haemogenic endothelium is restricted to the 23GFP+EC population. (a) Experimental approach for data shown inFigs 2,3,4,5. (b) Generation of haematopoietic progeny by 23GFP+or 23GFP−VE-Cadh+Ter119−CD45−CD41−ECs from E8.5 (5–12 sp) concepti or E10.5 (29–35 sp) AGM+VU on OP9 stroma. Black arrowhead: round semi-adherent haematopoietic cells; white arrowhead: adherent cobblestone-like cells (scale bar, 50 μm). Flow cytometric analysis confirmed the presence of CD45+haematopoietic cells. Data are representative of at least three independent cocultures. (c) Representative flow cytometric analysis of haemogenic cultures demonstrates both B-lymphoid (CD19) and myeloid (Mac1 or Gr1) cell generation. (d) May-Grünwald Giemsa stained cytospins of haemogenic cultures reveal myeloid (arrowhead, and ii–iv) and blast-like (arrow and v) haematopoietic cells. Asterisks point out OP9 stromal cells. Scale bar, 10 μm. (e) 23GFP+or 23GFP−VE-Cadh+Ter119−CD45−CD41−cells were isolated from E8.5 (5–12 sp) conceptus or E10.5 (29–35 sp) AGM+VU, and cultured on OP9 stroma to support endothelial tubule formation. Tubules were visualized by CD31 staining after 4 days of culture. Representative images and quantification (mean±s.d.) of endothelial tubules generated in OP9 cocultures by 23GFP+or 23GFP−VE-Cadh+Ter119−CD45−CD41−cells isolated from E8.5 (5–12 sp) conceptus or E10.5 (29–35 sp) AGM+VU (n=3). Only very limited endothelial tubule formation was observed in the 23GFP+EC population at E10.5, shown is one of 11 tubules. Scale bar, 200 μm. Figure 2: Haemogenic endothelium is restricted to the 23GFP + EC population. ( a ) Experimental approach for data shown in Figs 2 , 3 , 4 , 5 . ( b ) Generation of haematopoietic progeny by 23GFP + or 23GFP − VE-Cadh + Ter119 − CD45 − CD41 − ECs from E8.5 (5–12 sp) concepti or E10.5 (29–35 sp) AGM+VU on OP9 stroma. Black arrowhead: round semi-adherent haematopoietic cells; white arrowhead: adherent cobblestone-like cells (scale bar, 50 μm). Flow cytometric analysis confirmed the presence of CD45 + haematopoietic cells. Data are representative of at least three independent cocultures. ( c ) Representative flow cytometric analysis of haemogenic cultures demonstrates both B-lymphoid (CD19) and myeloid (Mac1 or Gr1) cell generation. ( d ) May-Grünwald Giemsa stained cytospins of haemogenic cultures reveal myeloid (arrowhead, and ii–iv) and blast-like (arrow and v) haematopoietic cells. Asterisks point out OP9 stromal cells. Scale bar, 10 μm. ( e ) 23GFP + or 23GFP − VE-Cadh + Ter119 − CD45 − CD41 − cells were isolated from E8.5 (5–12 sp) conceptus or E10.5 (29–35 sp) AGM+VU, and cultured on OP9 stroma to support endothelial tubule formation. Tubules were visualized by CD31 staining after 4 days of culture. Representative images and quantification (mean±s.d.) of endothelial tubules generated in OP9 cocultures by 23GFP + or 23GFP − VE-Cadh + Ter119 − CD45 − CD41 − cells isolated from E8.5 (5–12 sp) conceptus or E10.5 (29–35 sp) AGM+VU (n=3). Only very limited endothelial tubule formation was observed in the 23GFP + EC population at E10.5, shown is one of 11 tubules. Scale bar, 200 μm. Full size image 23GFP + HE loses its endothelial potential during development As well as the expression of endothelial markers, the ability of cells to form endothelial tubules/sheets in OP9 culture is considered a hallmark of endothelial potential and function [10] , [11] , [29] , [32] , [33] . Analysis of endothelial tubule/network formation in OP9 cocultures supplemented with vascular endothelial growth factor showed that the E8.5 23GFP + and 23GFP − EC populations readily formed CD31 + vascular tubules and networks at an equal frequency ( Fig. 2e ). At E10.5, this capacity was severely reduced among the 23GFP + ECs, but maintained in the 23GFP − ECs. Although a few endothelial tubules/networks were detected in cultures of 23GFP + cells, these results challenged the concept of HE as a bona fide endothelial cell able to generate endothelial tubules or sheets while also giving rise to haematopoietic progeny [29] . To explore this directly, we performed clonal cultures of E8.5 to E10.5 HE. In these cultures, a single 23GFP + HE cell never had both haematopoietic and endothelial potential (over 1,800 single cells analysed; Table 1 ; Supplementary Fig. S2a ). Haematopoietic progeny and endothelial tubules were generated at frequencies comparable with those obtained in bulk and limiting dilution cultures, but never from the same cell ( cf . Fig. 2e and Supplementary Fig. S2e ). Importantly, in line with previous reports [5] , [10] , [29] , [34] , single E7.5 23GFP + mesodermal (Flk1 + VE-Cadh −/lo CD41 − ) cells plated in control experiments did give rise to both haematopoietic and endothelial cells, which indicates that our OP9 cultures can readout coexistence of haemogenic and endothelial potential in single cells ( Supplementary Fig. S3 ). In conclusion, the failure to detect haemogenic and endothelial potential in a single 23GFP + HE cell indicates that if this potential exists in these cells, it is exceedingly rare, lending no experimental support for the conventional model depicted in Fig. 3 . Instead, we observed that 23GFP + HE undergoes dynamic functional changes over time, showing an increased capacity to generate haematopoietic progeny, concomitant with an unexpected early decrease in endothelial potential ( Table 1 ; Fig. 3 ). Importantly, this loss of endothelial potential was missed in previous studies, presumably at least in part because without a tool such as the 23GFP mice, HE could not be separated from non-haemogenic ECs. Table 1 23GFP + HE undergoes dynamic functional changes early in development. 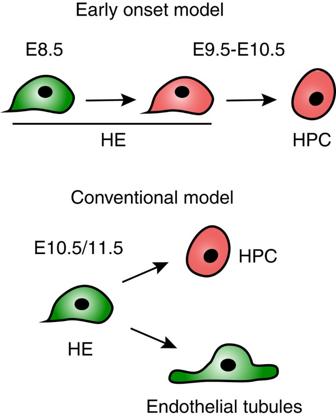Figure 3: Early onset model of EHT. In the conventional model of EHT (right side), haemogenic endothelium is considered as an endothelial cell capable of generating endothelial tubules and giving rise to haematopoietic progeny. This model is not supported by the functional data. In contrast, the data suggest an alternative model of EHT, with 23GFP+haemogenic endothelium undergoing an early onset of haematopoietic differentiation, and loss of endothelial potential. Full size table Figure 3: Early onset model of EHT. In the conventional model of EHT (right side), haemogenic endothelium is considered as an endothelial cell capable of generating endothelial tubules and giving rise to haematopoietic progeny. This model is not supported by the functional data. In contrast, the data suggest an alternative model of EHT, with 23GFP + haemogenic endothelium undergoing an early onset of haematopoietic differentiation, and loss of endothelial potential. Full size image 23GFP + HE expresses key haematopoietic and endothelial genes To begin to analyse the molecular mechanisms that underlie the functional changes of 23GFP + HE, we performed quantitative RT–PCR (qRT–PCR) on cells isolated from the E8.5 to E10.5 PAS/AGM+VU. As only few cells can be obtained from these tissues, we used the Fluidigm platform, which allows for the simultaneous analysis of multiple genes in small cell numbers. Genes coding for transcription factors affiliated with the haematopoietic lineage [35] , [36] were analysed on samples of 25 cells each, obtained from pooled tissues ( Fig. 4 ). Non-haemogenic ECs and emerging CD41 + HPCs isolated from the same embryos were analysed in parallel. Strikingly, genes coding for transcription factors associated with the early specification of the haematopoietic system such as Meis1, Gata2 , Gata3 and Tal1 (Scl) , were expressed at higher levels in 23GFP + HE than in non-haemogenic ECs. For Meis1, Gata2, and Gata3 this was apparent already at E8.5. From E9.25, the haematopoietic master regulator Runx1 was readily detected in the 23GFP + HE but not in the 23GFP − ECs. Expression of known Runx1 target genes such as Gfi1 (ref. 37 ) and Sfpi1 (Pu.1) [38] closely followed Runx1 expression in the HE. Other haematopoietic-affiliated genes (for example, Myb, a marker of hematopoietic commitment [39] ) also followed this pattern. Altogether, these results support a stepwise establishment of the haematopoietic programme in the 23GFP + HE starting already at E8.5. 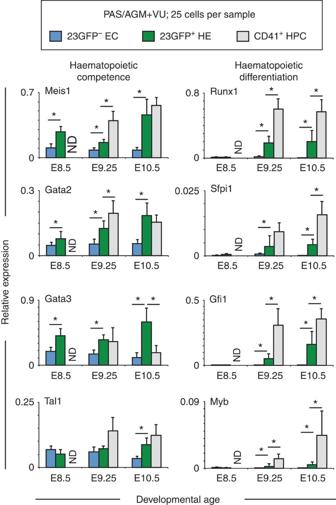Figure 4: Fluidigm qRT–PCR analysis of 23GFP+(green) and 23GFP−(blue) VE-Cadh+Ter119−CD45−CD41−ECs and/or VE-Cadh+Ter119−CD45−CD41+HPCs (grey) from E8.5 (5–9 sp), 9.25 (18-22 sp), and 10.5 (32–36 sp) PAS/AGM+VU. Data are normalized to the mean of the reference genesHprt1andBActand are the mean±s.d. of a total of 4–7 pools of 25 cells from two independent experiments. ND, not done. *P<0.05 (Student’st-test). Figure 4: Fluidigm qRT–PCR analysis of 23GFP + (green) and 23GFP − (blue) VE-Cadh + Ter119 − CD45 − CD41 − ECs and/or VE-Cadh + Ter119 − CD45 − CD41 + HPCs (grey) from E8.5 (5–9 sp), 9.25 (18-22 sp), and 10.5 (32–36 sp) PAS/AGM+VU. Data are normalized to the mean of the reference genes Hprt1 and BAct and are the mean±s.d. of a total of 4–7 pools of 25 cells from two independent experiments. ND, not done. * P <0.05 (Student’s t -test). Full size image Single-cell analysis reveals the transitory nature of HE To explore the dynamics of the haematopoietic commitment process at the single-cell level at which fate changes actually occur, we isolated 268 single 23GFP + HE from E8.5 to E11.5 PAS/AGM+VU ( Table 2 ) and performed single-cell Fluidigm qRT–PCR for 18 haematopoietic and endothelial-affiliated genes, including 10 core haematopoietic transcription factors [35] , [40] . Two hundred and eighty-five non-haemogenic ECs, 212 recently emerged CD41 + HPCs, and 38 more mature haematopoietic cells, referred to as CD45 + HPCs (23GFP + VE-Cadh + Ter119 − CD41 + CD45 + ) were analysed in parallel. Principal component analysis (PCA) revealed the relationships between all 803 individual cells ( Fig. 5a ). Non-haemogenic ECs (blue) and the CD45 + HPCs (yellow) formed two clearly distinct clusters along component 1. The endothelial genes Kdr , Tek and the haematopoietic genes Sfpi1, Myb, Runx1, Gfi1 and Itgb3 contributed most to the separation of these cell types. In contrast, CD41 + HPCs (red) were more scattered along component 1, indicating a continuum in maturation towards fully determined CD45 + HPCs (see also the E9.5 and E10.5 PCA plots in Supplementary Fig. S4a ). The 23GFP + HE cells (green) were scattered along component 1 and 2, showing increasing segregation from the non-haemogenic ECs and intermingling with CD41 + HPCs ( Fig. 5a ; Supplementary Fig S4a ), thus bearing out at the single-cell molecular level the dynamic functional changes observed in this transitory population over developmental time. Table 2 Number of single PAS/AGM+VU cells used in Fluidigm qRT–PCR analysis. 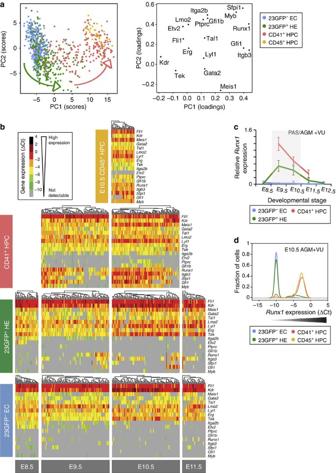Figure 5:Single-cell expression analysis reveals the transitory nature of 23GFP+HE. (a) Principal component projections of all 803 cells in the first and second components. Data represent all single cells, from all time points, analysed together. Individual cells were coloured retrospectively based on the phenotype they were sorted on. Arrows indicate the direction of maturation of 23GFP+HE cells (green) and CD41+HPC (red). (b) Heat maps showing the expression of the 18 endothelial- and haematopoietic-related genes in single cells for all cell types analysed. The data are ΔCtto the mean ofAtp5a1andUbcreference genes and colour coded as ΔCtsteps. Columns represent individual cells, displayed after hierarchical clustering so that similar expression profiles are closer together, and rows represent the individual genes ordered based on the hierarchical clustering of all data. (c) Narrow window ofRunx1expression in 23GFP+HE. Data are normalized to the mean of the reference genesHprt1andAtp5a1and are the mean±s.d. of a total of 4 to 6 pools of 25 cells from two independent experiments except E12.5 (one experiment with three pools of cells). E8.5 (6–13sp), E9.5 (19–26sp) and E10.5(32-38sp). (d) Kernel density plots of the single-cell data showing increasingRunx1levels in EC, HE and HPC at E10.5. Full size table Figure 5: Single-cell expression analysis reveals the transitory nature of 23GFP + HE. ( a ) Principal component projections of all 803 cells in the first and second components. Data represent all single cells, from all time points, analysed together. Individual cells were coloured retrospectively based on the phenotype they were sorted on. Arrows indicate the direction of maturation of 23GFP + HE cells (green) and CD41 + HPC (red). ( b ) Heat maps showing the expression of the 18 endothelial- and haematopoietic-related genes in single cells for all cell types analysed. The data are Δ C t to the mean of Atp5a1 and Ubc reference genes and colour coded as Δ C t steps. Columns represent individual cells, displayed after hierarchical clustering so that similar expression profiles are closer together, and rows represent the individual genes ordered based on the hierarchical clustering of all data. ( c ) Narrow window of Runx1 expression in 23GFP + HE. Data are normalized to the mean of the reference genes Hprt1 and Atp5a1 and are the mean±s.d. of a total of 4 to 6 pools of 25 cells from two independent experiments except E12.5 (one experiment with three pools of cells). E8.5 (6–13sp), E9.5 (19–26sp) and E10.5(32-38sp). ( d ) Kernel density plots of the single-cell data showing increasing Runx1 levels in EC, HE and HPC at E10.5. Full size image Analysis of gene expression on a per cell basis showed further similarities and differences between 23GFP + HE and 23GFP − ECs. At E8.5, both the 23GFP + HE and 23GFP − EC showed stochastic, low-level sampling [41] of genes associated with haematopoietic differentiation ( Runx1 , Gfi1 , Sfpi1 and c-Myb ). Moreover, both HE and non-haemogenic ECs widely expressed Itga2b (CD41) mRNA, a marker previously reported to be specific to HPCs [42] . After E8.5, Itga2b expression was undetectable in HE and non-haemogenic ECs, to be expressed again when cells develop into CD41 + /CD45 + HPCs. This unexpected [43] , [44] early endothelial expression of Itga2b was confirmed by CD41 immunofluorescence ( Supplementary Fig. S5a,b ), indicating that nascent endothelium of the PAS expresses low levels of CD41. We speculate that all nascent endothelium is competent to respond to haematopoiesis-inducing signals [45] . Evidence of haematopoietic development was however only seen among the 23GFP + HE cells, with ~50% of the E8.5 HE showing upregulation of the homeobox gene Meis1 , in line with the population data ( cf . Figs 4 and 5b ). Interestingly, this increased Meis1 (ref. 46 ) expression in HE was accompanied by a downregulation of Etv2 , an Ets transcription factor expressed in early endothelial cells [47] (E8.5, Fig. 5b , and see Supplementary Fig. S4b for the Pearson’s correlation analysis), suggestive of a previously unrecognized antagonistic relationship between Meis1 and Etv2 in establishing the haematopoietic programme. Meis1 (as well as Gata2 ) expression was maintained/increased in nearly all HE cells over developmental time, contributing to their segregation from the 23GFP − ECs ( Fig. 5b ). Thus, it appears that only the 23GFP + cells received and/or responded to haematopoiesis-inducing signals and have begun their journey along the haematopoietic lineage. Haematopoietic specification of HE initiates at E9.5 In the E9.5 PAS+VU, ~50% of the 23GFP + HE expressed the master haematopoietic regulator Runx1 ( Fig. 5b ). Only cells with the highest Runx1 levels co-expressed known Runx1 target genes such as Sfpi1 and Gfi1 , indicating the further unfolding of the haematopoietic programme. Correspondingly, these cells showed decreased Kdr (Flk1) expression, establishing at the single-cell level the reported antagonistic effect of Runx1 on Kdr [48] ( Fig. 5b ; and Supplementary Fig. S4b for Pearson’s correlation analysis). 23GFP + HE from the E10.5 AGM+VU also expressed Runx 1 and its downstream targets, albeit in fewer cells. Interestingly, Runx1 levels in HE peaked between E9.5 and E10.5 and decreased rapidly thereafter ( Fig. 5b,c ). As Runx1 is a critical regulator of the hematopoietic programme, this suggests that the initiation of the haematopoietic commitment process in HE, that is, the specification of the hematopoietic fate, occurs in a short burst. Never did we see any gene expression profile indicative of coordinated unfolding of the haematopoietic programme in 23GFP − cells, in line with their lack of haemogenic potential. In contrast, approximately half of the E9.5 CD41 + HPCs co-expressed Runx1 , Sfpi1 and/or Gfi1 (but not yet Myb ), indicative of a rapid transition of newly specified HE cells into the CD41 + pool, also seen from the overlap between these two cell types in PCA ( Fig. 5a ). The rapid changes in gene expression seen upon the induction of Runx1 in HE are consistent with the model where Runx1 orchestrates the assembly of a haematopoiesis-specific pattern of transcription factor binding [49] . Once the cells expressed CD41, they expressed higher levels of Runx1 and its direct targets, upregulated Myb [39] , Gfi1b [50] and Itgb3 (CD61 (ref. 43 )), and further downregulated Kdr , reflecting progressive locking in of the haematopoietic programme and development into fully determined CD45 + HPCs (E9.5 and E10.5, Fig. 5b–d and Supplementary Fig. S4b ). Here, we show that a transgenic GFP reporter expressed under the spatiotemporal control of the Runx1 +23 hematopoietic enhancer allows for the positive isolation of all haemogenic cells, from mesoderm as well as the major embryonic arteries of the mouse conceptus. We have used this model to begin to understand the molecular and temporal regulation of EHT at the clonal level. To our knowledge, our study is the first clonal functional and molecular analysis of embryonic HE undergoing EHT. Combined high-throughput single cell functional and transcriptional analysis allowed us to reveal that EHT is accompanied by an early loss of endothelial potential along with a gradual unfolding of the haematopoietic programme, as opposed to a segregation of haematopoietic and endothelial programmes in a single cell. Our data show that the process of commitment to the haematopoietic lineage, consisting sequentially of specification and determination of the hematopoietic programme, is first initiated at E9.5 in CD41 − 23GFP + HE, when these cells are still part of the endothelial wall. This observation places the CD41 − 23GFP + HE upstream of recently identified CD41 lo pre-HSCs [51] , [52] , and it will be of interest to assess the lineal relationship between the two. In conclusion, our results re-write the concept of haematopoietic specification during EHT and have important implications for the design of future experiments aimed at obtaining a mechanistic understanding of EHT, directing the search for key haematopoietic inducing signals and critical molecular pathways to earlier developmental time points than previously anticipated. This in turn impacts on the future generation of definitive haematopoietic stem and progenitor cells from embryonic stem/induced pluripotent cells or via direct reprogramming. Timed matings and embryo collection For timed pregnancies, (CBA × C57BL/6)/F1 females (6–26 weeks old) were mated overnight with 23GFP transgenic males (6–52 week old, maintained on a mixed (CBA × C57BL/6) background. Embryos were collected in phosphate-buffered saline (PBS; Gibco, Invitrogen) supplemented with 10% fetal calf serum (FCS; batch tested and obtained from either Biosera or PAA Laboratories), 50 U ml −1 penicillin, and 50 μg ml −1 streptomycin (Cambrex Corporation). E8.5 to E10.5 embryos were staged by counting somite pairs. 23GFP transgenic embryos were identified by fluorescence illumination (X-Cite 120; Improvision) on a Leica MZFLIII microscope. Mice were housed with free access to food and water. All procedures were in compliance with United Kingdom Home Office regulations and approved by the Ethical Review Committee of the Clinical School and the Home Office. Dissections and generation of cell suspensions E8.5 concepti and later stage yolk sac, PAS/AGM, VU vessels and were dissected in PBS supplemented with 10% FCS (batch tested and obtained from either Biosera or PAA Laboratories), 50 U ml −1 penicillin, and 50 μg ml −1 streptomycin (Cambrex Corporation) using watch makers forceps and 25 G needles. Concepti were dissected without the ectoplacental cone, and in part of the experiments without the head and heart region. Tissues were pooled and incubated for 20 min at 37 °C in PBS supplemented with 10% FCS, 50 U ml −1 penicillin, 50 μg ml −1 streptomycin and 0.12% (w/v) of collagenase (Type I, Sigma), and dissociated by pipetting. Suspensions were washed, and viable cells were counted on the basis of trypan blue (Sigma-Aldrich) exclusion using a Neubauer haemocytometer. Flow cytometry and cell sorting Embryonic cells were isolated by flow cytometry using a 100 μm nozzle at 30 p.s.i. and <1,500 events per second (MoFlow; Beckman Coulter). For single-cell qRT–PCR, cells were sorted directly using FACSAria III with an 85 μm nozzle (Becton Dickinson). Analysis was performed on CyAn ADP (Beckman Coulter). Antibody staining was carried out on ice and in the dark for 15 min in PBS supplemented with 10% FCS (batch tested and obtained from either Biosera or PAA Laboratories) and 50 U ml −1 penicillin, and 50 μg ml −1 streptomycin (Cambrex Corporation). Cells were collected into FCS-coated tubes and recounted prior to plating where possible. Antibodies and conjugates ( Supplementary Table S1 ) were titrated to determine their optimal concentration of use. Gates were defined using unstained, single stained and fluorescence minus onestained cells. Dead cells were excluded based on Hoechst 33258 (Invitrogen) uptake. Data were acquired and analysed using Summit (BC) or FACS Diva (BD) software. Fluorescent microscopy Embryos were fixed in 4% paraformaldehyde (Electron Microscopy Sciences) for 1–2 h at 4 °C, washed in PBS, and soaked in 15% (w/v) sucrose for 2–4 h at 4 °C. Samples were snap-frozen in Tissue-Tek OCT compound (Sakura, Siemens Medical Solutions Diagnostics) and sectioned at 10 μm on a Leica CM3050s cryostat, collected onto Superfrost plus glass slides (VWR) and after air drying, washed in PBS. For VE-Cadh or CD41 staining, sections were block permeated with 10% FCS in 0.05% Tween/PBS for 30 min at RT, incubated with purified rat anti-mouse VE-Cadh or CD41 antibody ( Supplementary Table S1 ) in 0.05% Tween PBS for 1 h at room temperature (RT), followed by 2 h incubation at RT with goat anti-rat AlexaFluor555 antibody (10 μg ml −1 ; Invitrogen) in 2% normal mouse serum and 0.05% Tween/PBS. For Runx1 Ab staining, sections were permeated with 1% Triton X-100/PBS for 10 min at RT, blocked with 10% FCS/PBS for 30 min at RT, incubated with polyclonal rabbit anti-mouse Runx1 antibody (kind gift of the Jessel lab) in 10% FCS/PBS overnight at 4 °C and stained for 2 h at RT with goat anti-rabbit AlexaFluor555 antibody (10 μg ml −1 ; Invitrogen) in 2% normal mouse serum and PBS. Slides were stained with TO-PRO-3 iodide (0.2 μM final concentration; Invitrogen) in PBS for 20 min, washed in PBS and coverslipped with Vectashield mounting medium containing 4′,6-diamidino-2-phenylindole (DAPI, Vector Laboratories). Sections were analysed and photographed with an Olympus BX51 camera (Olympus), Radiance 2000 Confocal Scanning System (Bio-Rad), and Laser Sharp 2000 software (Zeiss). Images were processed using Confocal Assistant 3.0 (CAS) and Adobe Photoshop (Adobe systems, Europe). Haematopoietic progenitor assay Colony-forming unit-culture (CFU-C) assays were performed using Methocult M3434 (Stem Cell Technologies). Cells were plated in duplicate in 35 mm culture dishes according to manufacturer’s instructions. Cultures were grown at 37 °C with 5% CO 2 with colonies scored after 7 days. OP9 maintenance OP9 cells (kindly provided by M. Yoder, Indianapolis) were maintained in αMEM (Gibco) with 20% defined FCS (Hyclone) and 0.22% sodium bicarbonate (Gibco) at 37 °C, 5% CO 2. Cells were passaged every 3 days using 0.05% Trypsin/EDTA (Gibco) at 37 °C for 6 min. For co-culture experiments, cells were resuspended in αMEM with 10% FCS and 1 × 10 −4 M 2-mercaptoethanol and plated at 23 × 10 3 cells per cm 2 24 h before the experiment. OP9 cocultures For single cell and limiting dilution cocultures, cells were directly sorted onto confluent OP9 stroma; for all other cocultures, cells were sorted and recounted prior to plating. Cocultures of OP9 with E7.5 cells were supplemented with 100 ng ml −1 SCF and grown for 5–7 days. For E8.5 to E10.5 haemogenic and single-cell assays, cultures were supplemented with 10 ng ml −1 IL7, 10 ng ml −1 SCF and 10 ng ml −1 Flt-3-ligand, and incubated for 8–10 days at 37 °C, 5% CO 2 . The haematopoietic nature of the cells generated in the OP9 cocultures was assessed by microscopy, flow cytometry and/or May-Grünwald Giemsa staining of cytospins. For endothelial assays, cells were cultured with 50 ng ml −1 recombinant murine vascular endothelial growth factor for 4 days at 37 °C 5% CO 2 . All cytokines were purchased from Peprotech ( Supplementary Table S2 ). To visualize endothelial cell growth, cultures were stained with rat anti-mouse CD31 (MEC13.3) followed by alkaline phosphatase-conjugated goat anti-rat and detected by Vectablue AP Substrate Kit III (Vector). Images were collected on an Olympus 1 × 51 microscope equipped with a Jenoptik ProgRes C14 camera, and processed using Adobe Photoshop. Microfluidic Quantitative RT–PCR Multiplex qRT–PCR was performed using the Fluidigm (Biomark) platform. TaqMan assays (Applied Biosystems; Supplementary Table S3 ) were pooled to a final concentration of 0.2 × . Cells were harvested directly into 10 μl RT-PreAmp Master Mix (consisting of 5 μl CellsDirect 2 × Reaction Mix (Invitrogen), 2.5 μl 0.2 × assay mix, 1.2 μl RT/Taq enzyme (CellsDirect qRT–PCR kit, Invitrogen), 1.2 μl TE buffer (Invitrogen) and 0.1 μl SUPERase-In (Ambion)). Collected samples were immediately vortexed and spun to aid cell lysis. Reverse transcription was performed at 50 °C for 15 min and inactivated at 95 °C for 5 min. In the same tube, cDNA was amplified by 22 cycles at 95 °C for 15 s followed by 60 °C for 4 min. The pre-amplified mix was immediately frozen at −20 °C until further analysis. Samples were diluted fivefold and analysed on 48.48 Dynamic Arrays according to manufacturers’ instructions, using the following PCR conditions: 95 °C for 10 min, followed by 40 cycles of 95 °C for 15 s and 60 °C for 1 min (Fluidigm, BioMark). Amplification curves were quality filtered using a threshold <0.65, and Ct thresholds were set for each assay with the same thresholds used across all experiments. Ct values were calculated by BioMark Real-time PCR Analysis software (Fluidigm). Data were exported to Excel as.csv files for subsequent analysis. Microfluidic quantitative RT–PCR analysis For population level analysis, two independent sorting experiments were performed each with 2–3 biological replicates of 25 cells. Data were analysed by the Δ C t method [53] , normalized to Hprt1 and BAct . For single-cell analysis, 20 haematopoietic and endothelial-affiliated genes and four housekeeping assays were analysed in duplicate with positive (20 cell) and negative (0 cell) controls analysed on each 48.48 array. Duplicate readings were averaged, and the data were filtered according to no template control reactions, (0 cell), and excluding C t >27. Genes that were not expressed were set to a C t of 27. All C t values were subtracted from the no template background of 27. Samples were included for downstream analysis based on the expression of Atp5a1 and Ubc with Δ C t values calculated using the mean Ct value of Atp5a1 and Ubc for each cell. Cdh5 and Cbfb assays were not used for single-cell analysis based on poor amplification curves. Hierarchical clustering, Pearson’s correlation and principal component analyses were performed in R ( http://www.r-project.org ) and did not include housekeeping genes. Microarray analysis Whole-genome expression analysis was performed using total RNA extracted using Trizol according to manufacturers’ instructions (Invitrogen) and purified using RNeasy Micro kit (Qiagen). With the same total amount of input RNA, triplicate samples were amplified with a WT-Ovation Pico RNA Amplification System followed by WT-Ovation cDNA Biotin Module V2 for cDNA labelling (NuGEN) and fragmentation, and were finally hybridized to Affymetrix Mouse Genome 430 2.0 arrays by standard protocols (Affymetrix) at the Stanford Protein and Nucleic Acid facility. The CEL files were normalized using RMA in the affy package [54] and a threshold of log expression value of 5 in at least one sample was used for selecting informative probes. Significantly differentially expressed genes were selected using the LIMMA [55] package with >1.0 absolute log fold change and adjusted (Benjamini Hockberg) P <0.05 for comparisons of HE versus E and HPC versus non-HPC samples. The union of these was then used to select probes for the heatmap generated by the gplots library ( http://www.CRAN.R-project.org/package=gplots ). Gene ontology enrichment analysis and annotation of the probe sets was done using Metacore ( http://www.thomsonreuters.com/metacore/ ), which uses the Multicore variation of the Fisher’s exact test and adjusts for multiple sample testing using FDR. Statistics Results, unless otherwise indicated, are expressed as mean±s.d. Two-tailed Student’s t -test was used to determine the level of significance with P<0.05 considered statistically significant and indicated by an asterisk. Accession codes: Microarray data have been deposited at GEO database under accession number GSE2075 . How to cite this article: Swiers, G. et al. Early dynamic fate changes in haemogenic endothelium characterized at the single-cell level. Nat. Commun. 4:2924 doi: 10.1038/ncomms3924 (2013).